C-terminal UBA domains protect ubiquitin receptors by preventing initiation of protein degradation The ubiquitin receptors Rad23 and Dsk2 deliver polyubiquitylated substrates to the proteasome for destruction. The C-terminal ubiquitin-associated (UBA) domain of Rad23 functions as a cis -acting stabilization signal that protects this protein from proteasomal degradation. Here, we provide evidence that the C-terminal UBA domains guard ubiquitin receptors from destruction by preventing initiation of degradation at the proteasome. We show that introduction of unstructured polypeptides that are sufficiently long to function as initiation sites for degradation abrogates the protective effect of UBA domains. Vice versa , degradation of substrates that contain an unstructured extension can be attenuated by the introduction of C-terminal UBA domains. Our study gains insight into the molecular mechanism responsible for the protective effect of UBA domains and explains how ubiquitin receptors can shuttle substrates to the proteasome without themselves becoming subject to proteasomal degradation. The sequence of events that results in the progressive degradation of proteins in the cytosolic and nuclear compartments of cells is tightly regulated and coordinated in a manner that limits the destructive action to designated substrates only, while leaving other proteins unharmed [1] . Protein substrates need to meet at least two requirements for efficient degradation to take place. The first prerequisite is that the substrates have to interact with the proteasome, a large barrel-shaped complex that harbours several proteolytic active subunits [2] . The canonical targeting signals for proteasomal degradation are Lys48-linked polyubiquitin chains that are typically conjugated to an internal lysine residue within the target protein [3] . A more recent study has revealed a second important requirement for degradation, namely, the presence of an unstructured initiation site that is essential to engage the unfolding machinery of the proteasome [4] . Although the compartmentalized nature of the proteasome provides an efficient way to confine proteolysis to proteins that are specifically targeted for degradation, it introduces at the same time some challenging constraints for substrates [5] . As the entrance of the proteasome particle can only accommodate passage of denatured polypeptide strands [6] , proteins need to be unfolded before they can be translocated into the proteolytic chamber of the proteasome [7] . The 19S regulatory particle of the proteasome is equipped with six AAA-ATPases that possess unfoldase activity and are located at the gate of the proteasome core particle [8] , [9] . To initiate the process of protein unfolding, the proteasome requires a loosely folded initiation site of at least 20–30 amino acids, from which it sequentially unfolds and hydrolyzes the protein [4] , [10] , [11] . In metazoan cells, the polyubiquitin-selective chaperone AAA-ATPase p97 Ufd1/Npl4 , which has a central role in ubiquitin-dependent proteasomal degradation [12] , is required for the degradation of folded substrates that lack an unstructured polypeptide, suggesting that this complex may be able to provide substrates with an unstructured initiation site before interaction with the proteasome [13] . The budding yeast ubiquitin receptors Rad23 and Dsk2 bind polyubiquitylated proteins with their ubiquitin-associated (UBA) domains and deliver these substrates to the proteasome for destruction [14] . Despite the fact that Rad23 and Dsk2 have to operate in close proximity to this proteolytic machinery, these proteins have long half-lives, suggesting that their polyubiquitylated cargo is selectively degraded by the proteasome, while the ubiquitin receptors themselves are left unharmed [15] , [16] . We have previously shown that the C-terminal UBA2 domain behaves as an intrinsic stabilization signal that protects Rad23 from proteasomal degradation [17] . Substitution of a critical leucine residue in the UBA2 domain causes Rad23 to be degraded in a manner that is dependent on its N-terminal ubiquitin-like (UbL) domain [17] , which is known to facilitate the interaction with the proteasome [16] . In this study, we have investigated, in detail, the protective effect of the UBA domains of Rad23 and Dsk2 with respect to the molecular mechanism that allows these ubiquitin receptors to function as reusable shuttles for delivering polyubiquitylated proteins to the proteasome. The UBA domain of Dsk2 functions as a stabilization signal Dsk2 shares with Rad23 not only its ability to deliver polyubiquitylated proteins to the proteasome [14] but also its long half-life [15] , [16] , which encouraged us to investigate whether the UBA domain of Dsk2 has a role in protecting this ubiquitin receptor from proteasomal degradation analogous to what has been observed for Rad23 (ref. 17 ). To this end, we substituted two conserved leucine residues in the UBA domain of Dsk2 for alanine residues in FLAG-tagged Dsk2 ( FLAG Dsk2 L368,369A ). Notably, structural analysis has revealed that the leucine at position 369 is part of a hydrophobic patch that is important for the typically tightly packed α-helical fold of UBA domains [18] , and simultaneous substitution of these two adjacent leucine residues abolishes ubiquitin binding [19] . These amino-acid substitutions resulted in a strongly reduced steady-state level of the mutant protein, as compared with its wild-type counterpart ( Fig. 1a ). To test whether the reduced steady-state levels of FLAG Dsk2 L368,369A were due to proteasomal degradation, we administrated the proteasome inhibitor MG132 to the yeast in a specific medium that allows efficient uptake of this compound [20] . Inhibitor treatment caused a striking accumulation of FLAG Dsk2 L368,369A , in line with efficient proteasomal degradation being responsible for the reduced levels ( Fig. 1a ). FLAG Dsk2 L368,369A had a short half-life ( Fig. 1b ) and was stabilized by administration of proteasome inhibitor, consistent with efficient proteasomal degradation of the mutant Dsk2 ( Fig. 1c ). Importantly, deletion of the UbL domain also resulted in stabilization of the mutant Dsk2, demonstrating that its degradation is largely dependent on its proteasome-interacting domain ( Fig. 1b ). 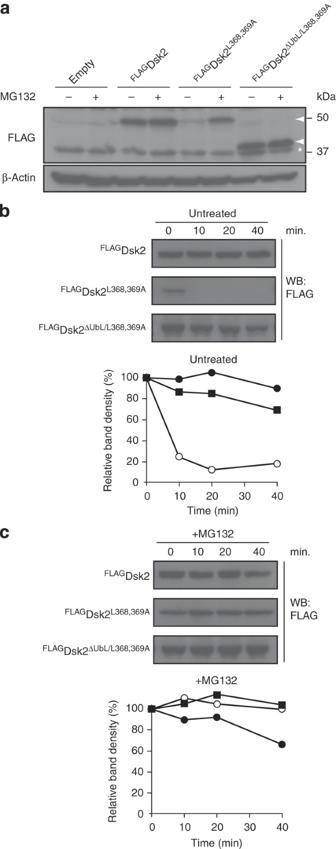Figure 1: The UBA domain of Dsk2 functions as a stabilization signal. (a) Steady-state levels of FLAG-tagged Dsk2 determined by western blotting with a FLAG-specific antibody.FLAGDsk2,FLAGDsk2L368,369AandFLAGDsk2ΔUbL/L368,369Awere ectopically expressed from a GAL1 promoter. Yeast was grown until early log phase. Wherever indicated, proteasome inhibitor was added to a final concentration of 50 μM, 2 h before harvesting. β-Actin is shown as loading control. Molecular weight markers are indicated. Asterisk marks a non-specific band. (b) Turnover ofFLAGDsk2 (closed circles),FLAGDsk2L368,369A(open circles) andFLAGDsk2ΔUbL/L368,369A(closed squares). Samples were taken at the indicated time points and probed with a FLAG-specific antibody. Densitometric quantification of the western blot is shown. (c) Turnover ofFLAGDsk2 (closed circles),FLAGDsk2L368,369A(open circles) andFLAGDsk2ΔUbL/L368,369A(closed squares) in the presence of 50 μM proteasome inhibitor MG132, as shown inb. Figure 1: The UBA domain of Dsk2 functions as a stabilization signal. ( a ) Steady-state levels of FLAG-tagged Dsk2 determined by western blotting with a FLAG-specific antibody. FLAG Dsk2, FLAG Dsk2 L368,369A and FLAG Dsk2 ΔUbL/L368,369A were ectopically expressed from a GAL1 promoter. Yeast was grown until early log phase. Wherever indicated, proteasome inhibitor was added to a final concentration of 50 μM, 2 h before harvesting. β-Actin is shown as loading control. Molecular weight markers are indicated. Asterisk marks a non-specific band. ( b ) Turnover of FLAG Dsk2 (closed circles), FLAG Dsk2 L368,369A (open circles) and FLAG Dsk2 ΔUbL/L368,369A (closed squares). Samples were taken at the indicated time points and probed with a FLAG-specific antibody. Densitometric quantification of the western blot is shown. ( c ) Turnover of FLAG Dsk2 (closed circles), FLAG Dsk2 L368,369A (open circles) and FLAG Dsk2 ΔUbL/L368,369A (closed squares) in the presence of 50 μM proteasome inhibitor MG132, as shown in b . Full size image Different stabilizing potentials of UBA and UIM domains More recently, it has been shown that a ubiquitin-interacting motif (UIM) in the transcription factor Met4, whose activity is regulated in a non-proteolytic manner [21] by the conjugation of Lys48-linked polyubiquitin chains [22] , prevents proteasomal degradation of Met4 (ref. 23 ). It has been proposed that the UIM domain protects Met4 by inhibiting ubiquitin chain assembly, allowing only formation of polyubiquitin chains that are below the critical length required for proteasomal degradation [23] . To test whether a similar phenomenon could be responsible for the protective effect of UBA domains, we compared the effects of the wild-type UBA2 domain and the mutant UBA2 L392A domain, which lacks protective activity [17] , on ubiquitylation of a well-characterized N-end rule green fluorescent protein (GFP) substrate, ubiquitin–arginine–GFP (Ub-R-GFP) [24] , [25] . Ubi-quitylated proteins were precipitated under reducing conditions to avoid contaminations with polyubiquitylated proteins bound to the UBA domain. We observed a very similar polyubiquitylation pattern for the reporter substrates, irrespective of the nature of the UBA domain ( Fig. 2a ). As the polyubiquitylation pattern was comparable in substrates carrying either the protective or mutant UBA domain, inhibition of ubiquitin chain elongation cannot fully explain the ability of UBA domains to protect substrates from proteasomal degradation. 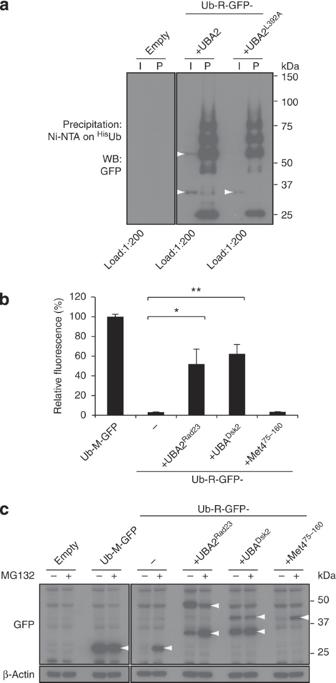Figure 2: Different stabilizing potentials of UBA and UIM domains. (a) Ub-R-GFP-UBA2 and Ub-R-GFP-UBA2L392Awere expressed in yeast together with His-tagged ubiquitin. Ubiquitylated proteins were precipitated using Ni beads and probed with a GFP-specific antibody. Input (I) and precipitated (P) samples are shown. Ub-R-GFP-UBA2 and Ub-R-GFP-UBA2L392Aare indicated. Note that the upper band in the Ub-R-GFP-UBA2 corresponds with diubiquitylated Ub-R-GFP-UBA2. Molecular weight markers are indicated. (b) Relative fluorescence levels of yeast expressing the Ub-M-GFP, Ub-R-GFP, Ub-R-GFP-UBA2Rad23, Ub-R-GFP-UBADsk2and Ub-R-GFP-UIMMet4analysed by flow cytometry. Ub-M-GFP was standardized as 100%. Values are means and standard deviations (n=3). *P<0.05, **P<0.01 (Student'st-test). (c) Western blot analysis with GFP-specific antibody of steady-state levels of Ub-M-GFP, Ub-R-GFP, Ub-R-GFP-UBA2Rad23, Ub-R-GFP-UBADsk2and Ub-R-GFP-UIMMet4in the absence or presence of 50 μM proteasome inhibitor MG132. Note that the upper bands correspond with diubiquitylated Ub-R-GFP-UBA2Rad23and putative monoubiquitylated Ub-R-GFP-UBADsk2. β-Actin is shown as loading control. Molecular weight markers are indicated. Specific bands are indicated with arrowheads. Figure 2: Different stabilizing potentials of UBA and UIM domains. ( a ) Ub-R-GFP-UBA2 and Ub-R-GFP-UBA2 L392A were expressed in yeast together with His-tagged ubiquitin. Ubiquitylated proteins were precipitated using Ni beads and probed with a GFP-specific antibody. Input (I) and precipitated (P) samples are shown. Ub-R-GFP-UBA2 and Ub-R-GFP-UBA2 L392A are indicated. Note that the upper band in the Ub-R-GFP-UBA2 corresponds with diubiquitylated Ub-R-GFP-UBA2. Molecular weight markers are indicated. ( b ) Relative fluorescence levels of yeast expressing the Ub-M-GFP, Ub-R-GFP, Ub-R-GFP-UBA2 Rad23 , Ub-R-GFP-UBA Dsk2 and Ub-R-GFP-UIM Met4 analysed by flow cytometry. Ub-M-GFP was standardized as 100%. Values are means and standard deviations ( n =3). * P <0.05, ** P <0.01 (Student's t -test). ( c ) Western blot analysis with GFP-specific antibody of steady-state levels of Ub-M-GFP, Ub-R-GFP, Ub-R-GFP-UBA2 Rad23 , Ub-R-GFP-UBA Dsk2 and Ub-R-GFP-UIM Met4 in the absence or presence of 50 μM proteasome inhibitor MG132. Note that the upper bands correspond with diubiquitylated Ub-R-GFP-UBA2 Rad23 and putative monoubiquitylated Ub-R-GFP-UBA Dsk2 . β-Actin is shown as loading control. Molecular weight markers are indicated. Specific bands are indicated with arrowheads. Full size image We next compared side-by-side the protective effects of the UBA2 domain of Rad23, the UBA domain of Dsk2 and the UIM of Met4 in the context of the Ub-R-GFP reporter substrate. For the latter, we used a fragment of Met4 consisting amino acids 75–160 (Met4 75–160 ), which includes the earlier identified UIM [23] and has been shown to be able to inhibit proteasomal degradation [26] . In striking contrast to the UBA domains, the UIM Met4 had no effect on the stability of the N-end rule reporter substrate. The low steady-state level of the reporter carrying the UIM Met4 was a result of efficient proteasomal degradation, as demonstrated by flow cytometric ( Fig. 2b ) and western blot analysis ( Fig. 2c ) of yeast expressing the fusions in the absence or presence of proteasome inhibitor. The differences of the protective effects of the UBA domains and the Met4 UIM in the context of the N-end rule reporter substrate suggest that divergent molecular mechanisms are responsible for the ability of these ubiquitin-binding domains to protect proteins from proteasomal degradation. A C-terminal UBA1 domain does not protect from degradation The protective UBA domains of Rad23 and Dsk2 are localized at the C termini of these proteins. We wondered whether the positioning of the UBA domains was of significance for their ability to protect substrates from proteasomal degradation. To address this issue, we swapped the internal UBA1 domain and C-terminal UBA2 domain within the Rad23 protein ( Fig. 3a ). We first replaced the C-terminal UBA2 domain with the UBA1 domain, giving rise to a Rad23 with two UBA1 domains (Rad23 UBA1/UBA1 ). Next, we replaced the internal UBA1 domain with the UBA2 domain to generate Rad23 UBA2/UBA1 , in which the two domains had been swapped. Expression of wild-type Rad23 UBA1/UBA2 , and the two variants Rad23 UBA1/UBA1 and Rad23 UBA2/UBA1 , in yeast revealed that the UBA1 domain is unable to protect even when placed at the same C-terminal position as the UBA2 domain ( Fig. 3b ). Furthermore, placing the UBA2 domain at the internal position inactivated its stabilizing potential, as evidenced by the efficient proteasomal degradation of the Rad23 UBA2/UBA1 variant. Taken together, there are two important conclusions from this experiment. First, it confirmed, now in the context of Rad23, our earlier conclusion [17] that the UBA1 domain is unable to function as a stabilization signal. Second, these data show that the UBA2 domain can only protect from proteasomal degradation when positioned at the C terminus, which corresponds with its native location. 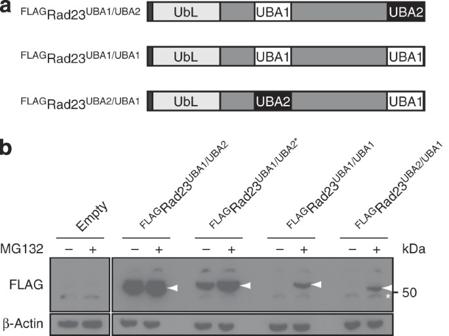Figure 3: A C-terminal UBA1 domain does not protect from degradation. (a) Schematic drawing of the positions of the UBA1 and UBA2 domains in wild-type Rad23 (Rad23UBA1/UBA2), Rad23UBA1/UBA1and Rad23UBA2/UBA1. (b) Steady-state levels of FLAG-tagged Rad23UBA1/UBA2(wild-type), Rad23UBA1/UBA2*(Rad23L392A), Rad23UBA1/UBA1and Rad23UBA2/UBA1were determined with a FLAG-specific antibody. Arrows indicateFLAGRad23 bands. β-Actin is shown as loading control. Molecular weight marker is indicated. Asterisk indicates a non-specific band. Figure 3: A C-terminal UBA1 domain does not protect from degradation. ( a ) Schematic drawing of the positions of the UBA1 and UBA2 domains in wild-type Rad23 (Rad23 UBA1/UBA2 ), Rad23 UBA1/UBA1 and Rad23 UBA2/UBA1 . ( b ) Steady-state levels of FLAG-tagged Rad23 UBA1/UBA2 (wild-type), Rad23 UBA1/UBA2* (Rad23 L392A ), Rad23 UBA1/UBA1 and Rad23 UBA2/UBA1 were determined with a FLAG-specific antibody. Arrows indicate FLAG Rad23 bands. β-Actin is shown as loading control. Molecular weight marker is indicated. Asterisk indicates a non-specific band. Full size image A conserved motif contributes to the protective effect We were intrigued by the fact that the UBA1 and UBA2 domains displayed such a striking difference in their ability to protect proteins from proteasomal degradation, despite their structural resemblance. Both domains adopt a fold with three tightly packed α-helix bundles in a conformation that is characteristic of UBA domains [27] . In an attempt to pinpoint the difference between the domains responsible for the divergent effects on proteasomal degradation, we generated chimeric UBA domains in which fragments containing the first, second and third helices from the UBA1 and UBA2 domains were combined ( Fig. 4a ). We found that most C-terminal helices of the UBA2 domain could be replaced with the equivalent fragment of the UBA1 domain, with only a modest impact on its protective effect, whereas the first and the second helices appeared to be more important for the stabilizing effect ( Fig. 4b ). Notably, the loop between the first two helices contains a highly conserved motif (Xaa-Gly-Phe/Tyr-Xaa) that is found to be important for specific binding events [27] as well as for ubiquitin-binding-assisted conformational switch [28] . We noticed that all protective UBA domains so far tested harboured a phenylalanine residue in this motif, whereas the UBA1 domains from Rad23 and the human homologue Rad23-A (hHR23A), which are both unprotective [17] , had a tyrosine residue at the same position ( Fig. 4c ). Remarkably, we found that replacing the tyrosine residue in this motif in the UBA1 domain with a phenylalanine residue resulted in a UBA1 domain that significantly increased the steady-state levels of the reporter substrate, although not to the same extent as the wild-type UBA2 domain ( Fig. 4d ). Turnover analysis showed that this single amino-acid substitution in the UBA1 domain indeed prolonged the half-life of the substrate ( Fig. 4e ). Our data suggest that the protective effect of the UBA2 domain is an intrinsic feature and identifies a well-conserved motif as a contributing factor. 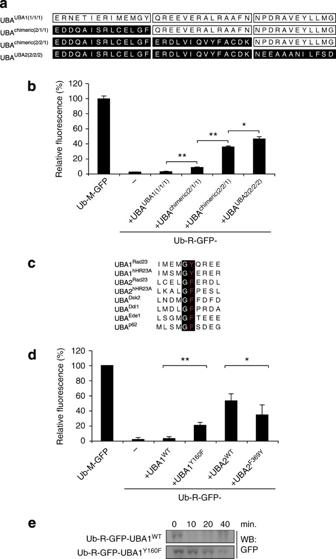Figure 4: A conserved motif contributes to the protective effect. (a) Schematic representation of the generation of chimeric UBA1/UBA2 domains. (b) Relative fluorescence levels of yeast cells expressing Ub-R-GFP with C-terminal UBA1, UBA2 and chimeric UBA domains analysed by flow cytometry. Values are means and standard deviations (n=3). *P<0.05, **P<0.01 (Student'st-test). (c) Alignment of the Xaa-Gly-Phe/Tyr-Xaa motif in the loop between helix 1 and helix 2 of a number of UBA domains. (d) Relative fluorescence levels of yeast cells expressing Ub-R-GFP-UBA1, Ub-R-GFP-UBA1Y160F, Ub-R-GFP-UBA2 and Ub-R-GFP-UBAF369Yanalysed by flow cytometry (the numbers refer to positions of these amino acids in Rad23). Values are means and standard deviations (n=6). *P<0.05, **P<0.01 (Student'st-test). (e) Turnover of Ub-R-GFP-UBA1 and Ub-R-GFP-UBA1Y160F. Samples were taken at the indicated time points and probed with a GFP-specific antibody. Figure 4: A conserved motif contributes to the protective effect. ( a ) Schematic representation of the generation of chimeric UBA1/UBA2 domains. ( b ) Relative fluorescence levels of yeast cells expressing Ub-R-GFP with C-terminal UBA1, UBA2 and chimeric UBA domains analysed by flow cytometry. Values are means and standard deviations ( n =3). * P <0.05, ** P <0.01 (Student's t -test). ( c ) Alignment of the Xaa-Gly-Phe/Tyr-Xaa motif in the loop between helix 1 and helix 2 of a number of UBA domains. ( d ) Relative fluorescence levels of yeast cells expressing Ub-R-GFP-UBA1, Ub-R-GFP-UBA1 Y160F , Ub-R-GFP-UBA2 and Ub-R-GFP-UBA F369Y analysed by flow cytometry (the numbers refer to positions of these amino acids in Rad23). Values are means and standard deviations ( n =6). * P <0.05, ** P <0.01 (Student's t -test). ( e ) Turnover of Ub-R-GFP-UBA1 and Ub-R-GFP-UBA1 Y160F . Samples were taken at the indicated time points and probed with a GFP-specific antibody. Full size image C-terminal unstructured polypeptides abrogate protection The importance of the C-terminal position of the UBA2 domain, combined with our earlier observation that the structural stability of mutant UBA domains of human p62 correlates with their protective effect [29] , raised the question of whether these domains can interfere with protein unfolding. Using designed substrates, it has previously been shown that proteasomes, when interacting with protein complexes, display a strong preference for those proteins that contain unstructured initiation sites [30] . Consistent with a critical role for preventing initiation of protein degradation, we found that introduction of a 34-amino-acid-long polypeptide, which is sufficiently long to function as an initiation site for proteasomal degradation [10] , [11] , strongly reduced the stabilizing effect of the UBA2 domain, resulting in low steady-state levels and accumulation of the reporter substrate in the presence of the proteasome inhibitor MG132 ( Supplementary Fig. S1 ). Promoter shut-off experiments showed that the half-life of the fusion harbouring the extension was substantially reduced ( Fig. 5a ). 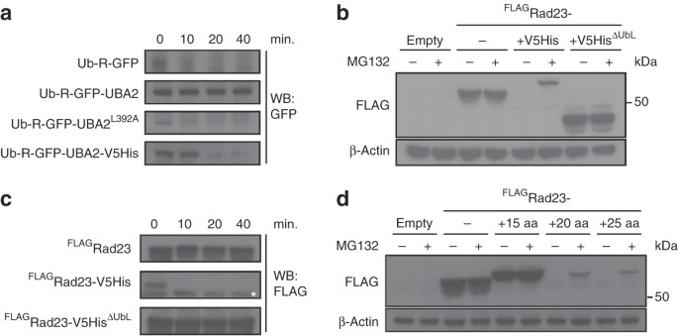Figure 5: C-terminal unstructured polypeptides abrogate protection. (a) Turnover of Ub-R-GFP, Ub-R-GFP-UBA2, Ub-R-GFP-UBA2L392Aand Ub-R-GFP-UBA2-V5His. Samples were taken at the indicated time points after switching off the expression and probed with a GFP-specific antibody. (b) Steady-state levels ofFLAGRad23,FLAGRad23-V5His andFLAGRad23-V5HisΔUbLin the absence or presence of the proteasome inhibitor MG132. β-Actin is shown as loading control. Molecular weight marker is indicated. (c) Turnover ofFLAGRad23,FLAGRad23-V5His andFLAGRad23-V5HisΔUbL. Samples were collected at the indicated time points and analysed with a FLAG-specific antibody. Asterisk indicates a non-specific band. (d) Steady-state levels ofFLAGRad23+15aa,FLAGRad23+20aa,FLAGRad23+25aa,FLAGRad23-V5His (33aa) andFLAGRad23-V5HisΔUbLin the absence or presence of the proteasome inhibitor MG132. The proteins were detected with a FLAG-specific antibody. β-Actin is shown as loading control. Molecular weight marker is indicated. Figure 5: C-terminal unstructured polypeptides abrogate protection. ( a ) Turnover of Ub-R-GFP, Ub-R-GFP-UBA2, Ub-R-GFP-UBA2 L392A and Ub-R-GFP-UBA2-V5His. Samples were taken at the indicated time points after switching off the expression and probed with a GFP-specific antibody. ( b ) Steady-state levels of FLAG Rad23, FLAG Rad23-V5His and FLAG Rad23-V5His ΔUbL in the absence or presence of the proteasome inhibitor MG132. β-Actin is shown as loading control. Molecular weight marker is indicated. ( c ) Turnover of FLAG Rad23, FLAG Rad23-V5His and FLAG Rad23-V5His ΔUbL . Samples were collected at the indicated time points and analysed with a FLAG-specific antibody. Asterisk indicates a non-specific band. ( d ) Steady-state levels of FLAG Rad23+15aa, FLAG Rad23+20aa, FLAG Rad23+25aa, FLAG Rad23-V5His (33aa) and FLAG Rad23-V5His ΔUbL in the absence or presence of the proteasome inhibitor MG132. The proteins were detected with a FLAG-specific antibody. β-Actin is shown as loading control. Molecular weight marker is indicated. Full size image We next investigated this phenomenon in the context of the native Rad23 protein and found that introduction of the C-terminal unstructured extension also converted the stable Rad23 to an efficiently degraded substrate of the proteasome ( Fig. 5b ). Importantly, degradation of Rad23 carrying the unstructured extension was dependent on its UbL domain ( Fig. 5b ). Whereas Rad23 remained stable over the 40-min time frame analysed, protein levels of the fusion carrying the unstructured extension were undetectable after 10 min ( Fig. 5c ). To investigate the minimal length requirement for the C-terminal extension, we truncated the 33 amino-acid-long unstructured polypeptide to generate fusion proteins with extensions consisting of 25, 20 and 15 amino acids. Whereas the 25 and 20 amino-acid-long extensions resulted in efficient proteasomal degradation of Rad23, the stability of the fusion carrying the 15 amino-acid-long extension was comparable with the stability of wild-type Rad23 ( Fig. 5d ). Thus, an extension consisting of at least 20 amino acids is required to facilitate proteasomal degradation, which corresponds with the minimal length requirement for unstructured initiation sites [10] , [11] . We conclude that introduction of C-terminal polypeptides that are sufficiently long to function as unstructured initiation sites abrogate the protective effect of the UBA2 domain. UBA domains can shield an internal unstructured polypeptide We observed that efficient proteasomal degradation of an UbL–GFP fusion ( Fig. 6a ) is strictly dependent on the presence of an unstructured polypeptide ( Fig. 6b,c ). Interestingly, positioning of the UBA2 domain at the C-terminal end of the extension resulted in a strong inhibition of proteasomal degradation of the UbL Rad23 fusion ( Fig. 6b,c ). Whereas the UBA2 domain blocked degradation of the fusion, the UBA1 domain did not have any noteworthy effect on its stability. Turnover experiments clearly showed that the C-terminal positioning of the UBA2 domain, but not the UBA1 domain, resulted in an extended half-life similar to the fusion that lacked an unstructured polypeptide ( Fig. 6d ). Similarly, we found that the UBA domain of Dsk2 protected the UbL Dsk2 –GFP carrying an unstructured polypeptide from proteasomal degradation ( Supplementary Fig. S2 ). The above data strongly suggest that UBA domains hinder the generation of an unstructured initiation site for degradation and provide an explanation for the importance of the C-terminal position for UBA-mediated protection from proteasomal degradation. 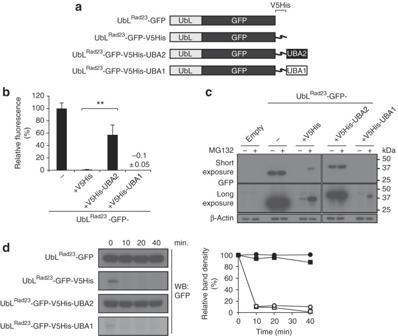Figure 6: C-terminal UBA domains of Rad23 can shield an internal unstructured polypeptide. (a) Schematic drawing of the UbLRad23-GFP fusions. (b) Flow cytometric quantification of the mean fluorescence intensities of yeast expressing UbLRad23-GFP, UbLRad23-GFP-V5His, UbLRad23-GFP-V5His-UBA2 and UbLRad23-GFP-V5His-UBA1. UbLRad23GFP was standardized as 100%. Values are means and standard deviations (n=3). **P<0.01 (Student'st-test). (c) Steady-state levels of UbLRad23-GFP, UbLRad23-GFP-V5His, UbLRad23-GFP-V5His-UBA2 and UbLRad23-GFP-V5His-UBA1 in the absence or presence of the proteasome inhibitor MG132. β-Actin is shown as loading control. Molecular weight markers are indicated. (d) Turnover of UbLRad23-GFP (closed circles), UbLRad23-GFP-V5His (open circles), UbLRad23-GFP-V5His-UBA2 (closed squares) and UbLRad23-GFP-V5His-UBA1 (open squares). Samples were collected at the indicated time points and probed with a GFP-specific antibody. Densitometric quantification of the blot is shown to the right. Figure 6: C-terminal UBA domains of Rad23 can shield an internal unstructured polypeptide. ( a ) Schematic drawing of the UbL Rad23 -GFP fusions. ( b ) Flow cytometric quantification of the mean fluorescence intensities of yeast expressing UbL Rad23 -GFP, UbL Rad23 -GFP-V5His, UbL Rad23 -GFP-V5His-UBA2 and UbL Rad23 -GFP-V5His-UBA1. UbL Rad23 GFP was standardized as 100%. Values are means and standard deviations ( n =3). ** P <0.01 (Student's t -test). ( c ) Steady-state levels of UbL Rad23 -GFP, UbL Rad23 -GFP-V5His, UbL Rad23 -GFP-V5His-UBA2 and UbL Rad23 -GFP-V5His-UBA1 in the absence or presence of the proteasome inhibitor MG132. β-Actin is shown as loading control. Molecular weight markers are indicated. ( d ) Turnover of UbL Rad23 -GFP (closed circles), UbL Rad23 -GFP-V5His (open circles), UbL Rad23 -GFP-V5His-UBA2 (closed squares) and UbL Rad23 -GFP-V5His-UBA1 (open squares). Samples were collected at the indicated time points and probed with a GFP-specific antibody. Densitometric quantification of the blot is shown to the right. Full size image Protective UBA domains cannot function as initiation sites Our observations that Rad23 variants, in which the C-terminal UBA2 domain has been mutated, are subjected to proteasomal degradation suggest that mutant UBA domains not only fail to protect but can also function as initiation sites. We tested this possibility by providing the UbL Rad23 –GFP with the UBA2 or UBA2 L392A domain of Rad23 and the UbL Dsk2 –GFP with the UBA or UBA L368,369A of Dsk2 ( Fig. 7a ). Consistent with this model, we found by flow cytometric ( Fig. 7b ) and western blot analysis ( Fig. 7c,d ) that the UBA domains could be clearly divided into two groups: (i) the mutant UBA2 L392A and UBA L368,369A domains, which facilitated degradation of the UbL-targeted proteins, and (ii) the protective UBA domains of Rad23 and Dsk2, which did not cause degradation of UbL-targeted proteins. These findings suggest that protective UBA domains prevent protein degradation through their inability to function as unstructured initiation sites for protein degradation. 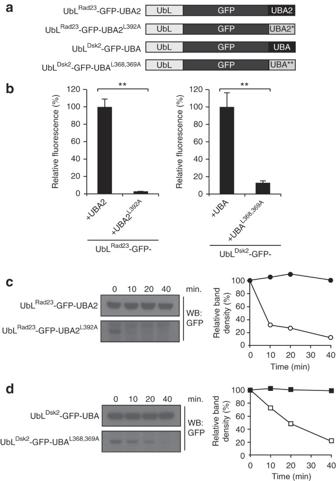Figure 7: Protective UBA domains cannot function as initiation sites. (a) Schematic drawing of the UbL-GFP fusions. (b) Flow cytometric quantification of the mean fluorescence intensities of yeast expressing UbLRad23-GFP-UBA2, UbLRad23-GFP-UBA2L392A, UbLDsk2-GFP-UBA or UbLDsk2-GFP-UBAL368,369A. UbLRad23-GFP-UBA2 and UbLDsk2-GFP-UBA were standardized as 100%. Values are means and standard deviations (n=3). **P<0.01 (Student'st-test). (c) Turnover of UbLRad23GFP-UBA2 (closed circles) and, UbLRad23GFP-UBA2L392A(open circles). Samples were collected at the indicated time points and detected with a GFP-specific antibody. Densitometric quantification of the blot is shown to the right. (d) Turnover of UbLDsk2-GFP-UBA (closed squares) and UbLDsk2-GFP-UBAL368,369A(open squares). Samples were collected at the indicated time points and analysed by western blotting with a GFP-specific antibody. Densitometric quantification of the blot is shown to the right. Figure 7: Protective UBA domains cannot function as initiation sites. ( a ) Schematic drawing of the UbL-GFP fusions. ( b ) Flow cytometric quantification of the mean fluorescence intensities of yeast expressing UbL Rad23 -GFP-UBA2, UbL Rad23 -GFP-UBA2 L392A , UbL Dsk2 -GFP-UBA or UbL Dsk2 -GFP-UBA L368,369A . UbL Rad23 -GFP-UBA2 and UbL Dsk2 -GFP-UBA were standardized as 100%. Values are means and standard deviations ( n =3). ** P <0.01 (Student's t -test). ( c ) Turnover of UbL Rad23 GFP-UBA2 (closed circles) and, UbL Rad23 GFP-UBA2 L392A (open circles). Samples were collected at the indicated time points and detected with a GFP-specific antibody. Densitometric quantification of the blot is shown to the right. ( d ) Turnover of UbL Dsk2 -GFP-UBA (closed squares) and UbL Dsk2 -GFP-UBA L368,369A (open squares). Samples were collected at the indicated time points and analysed by western blotting with a GFP-specific antibody. Densitometric quantification of the blot is shown to the right. Full size image Our data strongly suggest that C-terminal UBA domains protect ubiquitin receptors from proteasomal degradation by preventing the generation of initiation sites for degradation, which are required for proper engagement of the inherent unfolding machinery of the proteasome [4] ( Fig. 8 ). The molecular mechanism that is proposed in this study is fundamentally different from the inhibition of ubiquitin chain elongation by which the UIM domain has been suggested to protect Met4 from degradation [23] . The implication of distinct mechanisms may seem surprising given that the UIM and UBA domain are structurally unrelated and have little in common except for their ability to selectively bind polyubiquitin chains. However, it is noteworthy that several properties of the involved proteins already argued against a shared mode of action. First, whereas the UIM prevents binding of Met4 to the proteasome [23] , Rad23 and Dsk2 need to physically interact with the proteasome in order to deliver their polyubiquitylated cargo [14] . Second, the UbL domains of Rad23 and Dsk2 bind directly to the Rpn1 subunit of the proteasome without the need for polyubiquitin modifications [31] , [32] , suggesting that blocking of polyubiquitylation will be inadequate to prevent binding of Rad23 and Dsk2 to the proteasome. Third, we recently showed that the structural stability rather than the ubiquitin binding properties of UBA domains is a critical determinant for their ability to protect from proteasomal degradation [29] . Fourth, the UBA domains in Rad23 and Dsk2 bind polyubiquitylated proteins designated for delivery at the proteasome [14] , which is hard to reconcile with a role of the very same domains in preventing proteasomal degradation by inhibiting ubiquitylation of the ubiquitin receptors themselves, as this would require simultaneous binding of ubiquitin chains conjugated to the ubiquitin receptor (to prevent chain elongation) and polyubiquitylated proteins (for delivery to the proteasome). 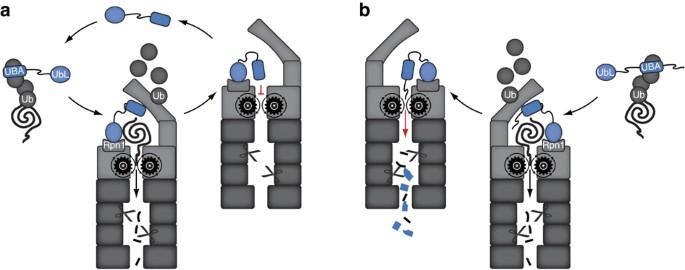Figure 8: Model for UBA-mediated protection from proteasomal degradation. (a) The schematic drawing shows an ubiquitin receptor (Rad23/Dsk2) that delivers a ubiquitylated substrate to the 26S proteasome. The ubiquitin receptor binds the proteasome through its N-terminal UbL domain that directly interacts with the Rpn1 subunit of the proteasome, thereby delivering the polyubiquitylated substrate bound to the UBA domain. Wild-type Rad23/Dsk2 contains a C-terminal UBA domain that resists initiation of protein degradation, resulting in release of the ubiquitin receptor from the proteasome. (b) In case the ubiquitin receptor has a mutant UBA domain or is provided with a polypeptide that can function as an unstructured initiation site, the ubiquitin receptor itself is translocated into the proteasome and hydrolyzed in the proteolytic chamber. Figure 8: Model for UBA-mediated protection from proteasomal degradation. ( a ) The schematic drawing shows an ubiquitin receptor (Rad23/Dsk2) that delivers a ubiquitylated substrate to the 26S proteasome. The ubiquitin receptor binds the proteasome through its N-terminal UbL domain that directly interacts with the Rpn1 subunit of the proteasome, thereby delivering the polyubiquitylated substrate bound to the UBA domain. Wild-type Rad23/Dsk2 contains a C-terminal UBA domain that resists initiation of protein degradation, resulting in release of the ubiquitin receptor from the proteasome. ( b ) In case the ubiquitin receptor has a mutant UBA domain or is provided with a polypeptide that can function as an unstructured initiation site, the ubiquitin receptor itself is translocated into the proteasome and hydrolyzed in the proteolytic chamber. Full size image The ubiquitin receptors Rad23 and Dsk2 are central players in ubiquitin-dependent proteasomal degradation since they, together with a few other substrate adaptors, are responsible for the delivery of polyubiquitylated substrates to the proteasome [33] . The question remains if a similar protective effect is also involved in rescuing other ubiquitin receptors from proteasomal degradation. The ubiquitin-binding subunit Rpn10, which is an integral part of the 19S regulator and important for the structural integrity of this complex [34] , is of particular interest as it carries a C-terminal UIM motif [35] , similar to the domain that protects Met4 from proteasomal degradation [23] . While our data show that Met4's UIM, unlike the protective UBA domains, is unable to safeguard reporter substrates from proteasomal degradation, it is difficult to directly extrapolate these findings to Rpn10. Although a recent report provided evidence that Rpn10 is polyubiquitylated and degraded by the proteasome [36] , which would support the idea that the UIM domain lacks a protective effect, we feel that further research is required as it can presently not be excluded that a possible protective effect of the UIM is regulated and becomes only apparent under specific conditions. Indeed, only recently has been found that Rpn10 is monoubiquitylated in a UIM-dependent manner and that this modification is important for its role in protein degradation [37] , suggesting that the interplay between ubiquitylation and Rpn10 may be more complicated than originally anticipated. An intriguing finding remains the observation that the internal UBA1 domain of Rad23 is unable to protect from proteasomal degradation [17] , even when positioned at the C terminus of Rad23, despite the fact that it shares its structural conformation [27] and its ability to bind ubiquitin [38] with the protective UBA2 domain. We found that a previously identified conserved motif [27] , which is present in the loop between the first two helices, partly determines the ability of the UBA2 domain to prevent degradation. Interestingly, it has been previously shown that this motif is not only involved in ubiquitin binding but also explains the selective binding of several proteins to the UBA2 domain of hHR23A [39] , [40] , [41] . Although ubiquitin binding is not a critical determinant for the protective effect [29] , our data do not exclude a contributing role for binding of ubiquitin or other proteins to UBA domains. In this respect, it is noteworthy that the UBA2 domain of hHR23A is able to bind two Lys48-linked ubiquitin molecules simultaneously, resulting in a structure in which the ubiquitin-binding domain is sandwiched in between two ubiquitin monomers [42] . It is feasible that the closed conformation of this complex may further hinder the unfolding by either stabilizing the structure or by making the C terminus of the UBA domain less accessible for the unfoldase machinery. Moreover, UBA domains can prevent ubiquitin chain elongation [43] , [44] and our data are compatible with a contributing role for this mode of action in particular, as sufficiently long polyubiquitin chains may otherwise allow the polyubiquitin-dependent chaperone p97/Cdc48 Ufd1/Npl4 complex to assist in protein unfolding by generating alternative initiation sites [13] . It is intriguing that the UIM and UBA domains target two independent events that are both critically required for efficient proteasomal degradation. The distinct roles of the transcription factor Met4 and the ubiquitin receptors Rad23 and Dsk2, respectively, may provide a plausible explanation for why these two steps are targeted by the respective domains. The modification with Lys48-linked polyubiquitin chains of Met4 regulates its activity in a non-proteolytic manner without implicating the proteasome [21] , [22] ; hence, preventing Met4 from interacting with the proteasome appears to be an efficient and robust way to avoid its degradation. On the contrary, Rad23 and Dsk2 need to interact with the proteasome in order to deliver their cargo [14] , making any type of interference with proteasome binding incompatible with their role in ubiquitin-dependent proteolysis. Instead, our data suggest that these proteins are shielded from the destructive activities of the proteasome by elements that prevent the initiation of degradation, a mechanism that is compatible with the observed transient interactions of ubiquitin receptors with the proteasome. The demonstration of divergent actions, targeting both substrate recruitment and unfolding, that allow ubiquitin-binding domains to interfere with the degradation of their corresponding proteins, highlights the intricate interplay between these domains and ubiquitin-dependent proteolysis and opens new avenues to probe into the molecular mechanisms that distinguish the fates of proteasome-interacting proteins from those of substrates. Yeast strains and media The experiments were performed in haploid derivates of strain DF5 (lys2-801, leu2-3, -112, ura3-52, his3-Δ200, trp1-1). Yeast transformed with episomal plasmids with GAL1 promoters was grown successively in synthetic medium with glucose, raffinose and galactose as sole carbohydrate source. For proteasome inhibition experiments, synthetic medium with 0.1% proline as sole nitrogen source was used [20] . The cultures were supplemented with 0.003% SDS in early mid-log phase, before the proteasome inhibitor MG132 ( Z -Leu-Leu-Leu-CHO, Biomol) was added at an OD 600 of 0.6 for 2 h at a final concentration of 50 μM (ref. 20 ). Construction of plasmids Yeast expression plasmids were generated by PCR, amplifying the open reading frames from genomic yeast DNA and introducing flanking restriction sites, which were used for subcloning them into the yeast expression vectors pYES2 (2μ, URA3; Invitrogen) or pYES3 (2μ, TRP1; Invitrogen). All constructs were verified by DNA sequencing. Protein analysis Total protein extracts of cultures in mid-log phase were obtained by lysis and precipitation in trichloroacetic acid. For GAL1 promoter shut-off experiments, transcription and translation were arrested by adding glucose and cycloheximide (Sigma) to final concentrations of 2% and 1 mg ml −1 , respectively. Aliquots were taken at the indicated time points and total protein extracts were prepared. Samples were heated for 10 min at 95 °C, subjected to SDS-PAGE and analysed by western blotting. Flow cytometric analysis Cultures were grown in galactose until mid-log phase and subjected to flow cytometric analysis on a FACScalibur (Beckton & Dickinson). Data were analysed with CellQuest software. Western blot analysis Total lysates were separated by SDS-PAGE and transferred onto nitrocellulose membranes (PROTRAN; Schleicher & Schuell). The membranes were blocked in phosphate-buffered saline supplemented with 5% skim milk and 0.1% Tween-20 for 1 h. This was followed by probing the membranes with monoclonal antibodies mix (Roche) or polyclonal antibodies (Invitrogen) specific to GFP in a 1:2,000 dilution for 1 h or a monoclonal antibody specific to the FLAG epitope (M5; Sigma) in 1:2,000 dilution for 1 h. After subsequent washing steps and incubation with peroxidase-conjugated goat anti-mouse or anti-rabbit serum, respectively (GE Healthcare), the membranes were developed by enhanced chemiluminiscence (GE Healthcare). Detection of ubiquitylated proteins Total yeast lysates of cultures (200 OD 600 units) in mid-log phase expressing His-tagged ubiquitin were obtained by lysis and precipitation in NaOH and trichloroacetic acid. Binding to Ni-NTA beads (Qiagen) was performed under denaturing conditions in buffer A (6 M guanidinium chloride, 100 mM NaH 2 PO 4 , 20 mM imidazole, 10 mM Tris (pH 8.0) and 0.05% Tween20) at 4 °C for 16 h. After subsequent washing with buffer A and buffer C (8 M urea, 100 mM NaH 2 PO 4 , 10 mM Tris (pH 6.3) and 0.05% Tween20), the beads were eluted in 1% SDS at 65 °C for 10 min. The samples were next heated and subjected to SDS-PAGE for western blotting. How to cite this article: Heinen, C. et al . C-terminal UBA domains protect ubiquitin receptors by preventing initiation of protein degradation. Nat. Commun. 2:191 doi: 10.1038/ncomms1179 (2011).